Functionalized arrays of Raman-enhancing nanoparticles for capture and culture-free analysis of bacteria in human blood Detecting bacteria in clinical samples without using time-consuming culture processes would allow rapid diagnoses. Such a culture-free detection method requires the capture and analysis of bacteria from a body fluid, which are usually of complicated composition. Here we show that coating Ag-nanoparticle arrays with vancomycin (Van) can provide label-free analysis of bacteria via surface-enhanced Raman spectroscopy (SERS), leading to a ~1,000-fold increase in bacteria capture, without introducing significant spectral interference. Bacteria from human blood can be concentrated onto a microscopic Van-coated area while blood cells are excluded. Furthermore, a Van-coated substrate provides distinctly different SERS spectra of Van-susceptible and Van-resistant Enterococcus , indicating its potential use for drug-resistance tests. Our results represent a critical step towards the creation of SERS-based multifunctional biochips for rapid culture- and label-free detection and drug-resistant testing of microorganisms in clinical samples. Surface-enhanced Raman spectroscopy (SERS) has been employed for label-free sensing of bacteria, exploiting its tremendous enhancement in the Raman signal. A typical SERS-active substrate consists of arrays of nano-scaled metallic objects, for example, Ag nanoparticles and etch-pits on Ag surfaces, which can sustain surface plasmon polariton resonance and enhance the Raman signal of molecules on or near the substrate [1] , [2] , [3] . Recently, a type of SERS-active substrate with uniformly large and highly reproducible Raman-enhancing power has been developed by growing Ag nanoparticles on arrays of anodic aluminum oxide (AAO) nanochannels to take advantage of the sub-10-nm inter-particle gaps, which act as 'hot junctions' for creating the electromagnetic enhancement [4] . The high sensitivity and reproducibility of such a substrate—hereafter referred to as Ag/AAO–SERS substrate—facilitated the use of SERS for chemical/biological sensing applications [5] , [6] , [7] , [8] , [9] , [10] , [11] , [12] , [13] , [14] , [15] , [16] , [17] , [18] , [19] , [20] , [21] , [22] . SERS of various types of bacteria including Gram-positive, Gram-negative and mycobacteria have been acquired and the response of bacteria to antibiotics has been examined [21] . Therefore, this SERS-based in situ detection method has a good opportunity to help solve the problem faced by conventional biological assay that commonly requires the sample preparation time ranging from days for fast growing bacteria to weeks for slow growers. To take full advantage of SERS for detecting and monitoring of bacteria, it is desirable to develop methods to capture bacteria from water, saliva, phlegm or blood samples and to directly load them onto SERS-substrates. Additionally, the operation of such methods ought not to compromise its SERS-sensing capability. It is known that bacteria bind vancomycin (Van) via hydrogen bonds between the peptidoglycan on the bacterial cell wall and the carbonyl and amine groups of Van. Van-coated magnetic nanoparticles have been employed to capture bacteria in water [23] , [24] , [25] , [26] , [27] , [28] . A sensible question to ask is whether we can endow the Van-coated SERS substrates with the concurrent functionalities of bacterial capturing and sensing. Here we demonstrate that functionalization of the Ag/AAO–SERS substrates by Van can not only dramatically enhance their ability to capture bacteria in liquid but also significantly increase their SERS signal. Furthermore, such Van-coated Ag/AAO–SERS substrates can be used to differentiate Van-susceptible and Van-resistant strains of Enterococcus . 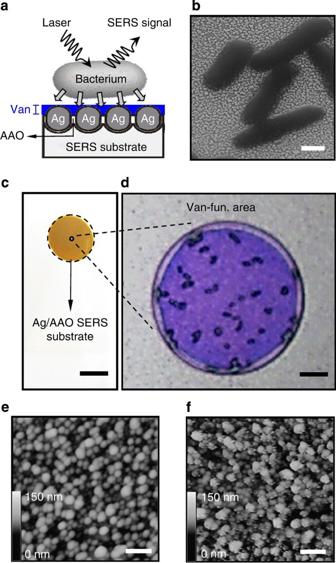Figure 1: Bacteria captured on Van-coated Ag/AAO–SERS substrate and AFM images showing the topography of Ag/AAO–SERS substrates. (a) Schematic diagram showing the cross-sectional view of a bacterium on a Van-coated substrate. (b) SEM image of bacteria on the substrate (scale bar, 500 nm). (c) Optical image of a substrate with a microscopic area (~30 μm) of Van coating (scale bar, 1 cm). (d) Optical image of the Van-coated region with the capturedE. coli(scale bar, 5 μm). (e) AFM image of the pristine substrate (scale bar, 300 nm) (f) AFM image of the Van-coated substrate (The streaky particles decorating the surface of Ag-nanoparticles are aggregates of Van. The streaks are most likely caused by the adhesion between the AFM tip and Van-aggregates; scale bar, 300 nm). Capture bacteria by Van-coated substrates Figure 1a shows schematically a bacterium on the capturing/sensing substrate prepared by immersing an Ag/AAO–SERS substrate into certain concentration (100 mM–80 μM) of Van hydrochloride aqueous solution for a fixed time period. To demonstrate its bacterium-capturing capability, one such substrate was immersed in a water sample with ultra-low concentration (10 2 cfu ml −1 ) of bacteria for 1 h and then rinsed in deionized water. The exemplified capture of Escherichia coli on the substrate was examined with scanning electron microscopy (SEM) and is displayed in Figure 1b . Because it is straightforward to coat a microscopic area on the Ag/AAO–SERS substrate by Van, using readily available microprinting technology such as inkjet printing, such substrate could also be used as a vehicle to concentrate bacteria in liquid samples including water and blood [29] . For example, as shown in Figure 1c,d , 30% of the bacteria in a 1-ml water sample—containing 10 2 cfu ml −1 of bacteria—were condensed onto a microscopic Van-coated area of 30 μm in diameter. The concentration of bacteria onto a microscopic area greatly reduces the laborious procedure required to locate the bacteria on the substrate and therefore facilitate their subsequent sensing by SERS. Figure 1: Bacteria captured on Van-coated Ag/AAO–SERS substrate and AFM images showing the topography of Ag/AAO–SERS substrates. ( a ) Schematic diagram showing the cross-sectional view of a bacterium on a Van-coated substrate. ( b ) SEM image of bacteria on the substrate (scale bar, 500 nm). ( c ) Optical image of a substrate with a microscopic area (~30 μm) of Van coating (scale bar, 1 cm). ( d ) Optical image of the Van-coated region with the captured E. coli (scale bar, 5 μm). ( e ) AFM image of the pristine substrate (scale bar, 300 nm) ( f ) AFM image of the Van-coated substrate (The streaky particles decorating the surface of Ag-nanoparticles are aggregates of Van. The streaks are most likely caused by the adhesion between the AFM tip and Van-aggregates; scale bar, 300 nm). Full size image Dependence of bacterium-capturing capability on Van-coating The bacterium-capturing capability of the Van-coated Ag/AAO–SERS is found to depend on the coverage of the Van coating, which is a function of the Van concentration in the solution used to coat the substrate. The coverage can be determined by the amount of Van left in the solution after the coating procedure (see details in the experimental section). To quantify the dependence of the capturing capability on the coverage of Van, the ratio between the number of bacteria ( Lactobacillus plantarum ) captured by a substrate with Van coating and that by a pristine substrate was determined. 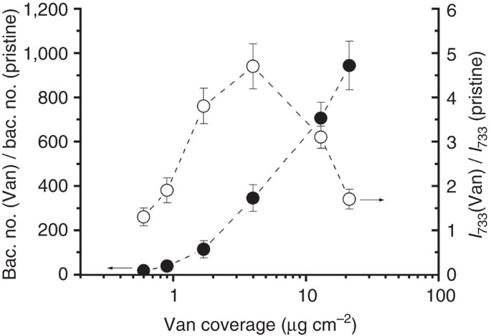Figure 2: Bacterium-sticking probability and SERS-sensing sensitivity of Van-coated substrate as a function of Van coverage. The number of bacteria captured on a Van-coated substrate is normalized by that on a pristine substrate to indicate its relative sticking probability, and the 733 cm−1SERS intensity ofL. plantarumon a Van-coated substrate is normalized by that on a pristine substrate to indicate its relative SERS sensitivity. Figure 2 shows that the ratio increases with increasing Van coverage and reaches a value as high as ~1,000 for a substrate with 20 μg cm −2 of Van coverage. The linear dependence of the capturing capability on the Van coverage raises many interesting questions about the interaction between Van and the molecules on the bacteria cell wall [30] , [31] , which could only be addressed properly after we have a better understanding of the cell-wall morphology of bacteria on Ag/AAO–SERS substrates with and without Van coating. Therefore, we defer the discussion until the morphological data are presented. Figure 2: Bacterium-sticking probability and SERS-sensing sensitivity of Van-coated substrate as a function of Van coverage. The number of bacteria captured on a Van-coated substrate is normalized by that on a pristine substrate to indicate its relative sticking probability, and the 733 cm −1 SERS intensity of L. plantarum on a Van-coated substrate is normalized by that on a pristine substrate to indicate its relative SERS sensitivity. 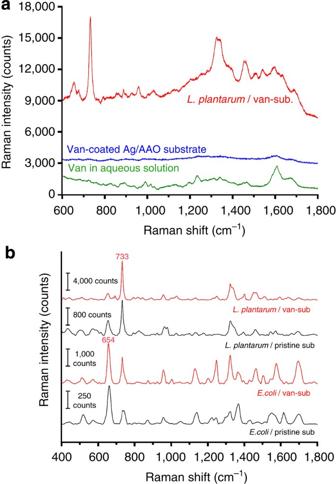Figure 3: SERS spectra ofL. plantarumandE. colion pristine and Van-coated SERS substrates. (a) Unprocessed SERS spectra ofL. plantarumon a Van-coated substrate prepared in 10−2M Van (Van coverage: 4 μg cm−2), and Raman spectra of such Van-coated substrate and Van in aqueous solution (5×10−2M). (b) Background-subtracted SERS spectra ofL. plantarumandE. colion pristine and Van-coated substrates. Full size image SERS of bacteria captured by Van-coated substrates Figure 3a shows the unprocessed SERS spectra of L. plantarum on a Van-coated substrate and that of such substrate itself. It clearly demonstrates that an adequate Van coating only introduces relatively low and broad features into the SERS spectrum of the captured bacteria, which can be easily removed by background–subtraction software programs. For comparison, the Raman spectrum of Van in water solution (5×10 −2 M) is also included in Figure 3a . It exhibits many sharp features below 1,500 cm −1 and 2 bands in the range between 1,500 and 1,700 cm −1 , which appear to be related to the two similar bands observed in the same region of the SERS spectrum for the Van-coated substrate. Similar sharp features remain on the SERS spectra of substrate prepared in dilute Van solution (6.4×10 −7 M); however, only broad bands survive on that prepared in dense solution (1×10 −2 M), as detailed in Supplementary Figure S1 . Figure 3: SERS spectra of L. plantarum and E. coli on pristine and Van-coated SERS substrates. ( a ) Unprocessed SERS spectra of L. plantarum on a Van-coated substrate prepared in 10 −2 M Van (Van coverage: 4 μg cm −2 ), and Raman spectra of such Van-coated substrate and Van in aqueous solution (5×10 −2 M). ( b ) Background-subtracted SERS spectra of L. plantarum and E. coli on pristine and Van-coated substrates. Full size image Candidates for the origin of the 1,300 cm −1 and 1,600 cm −1 broad bands include amide III (1,230 to 1,235 cm −1 ) [7] , [32] , carbohydrates (1,200 to 1,460 cm −1 ) [32] , carboxyl (1,600 to 1,609 cm −1 ) [32] , and C=O stretching (1,656 to 1,676 cm −1 ) [32] , [33] , [34] . Such featureless, broad spectral characteristics are likely caused by the spectral overlapping of inhomogeneously broadened vibrational signatures that are originated from the aggregate nature of Van. Van nanoparticles, few nanometers in size, are formed on the surface of the Van-coated Ag/AAO–SERS substrates prepared in the dense solution ( Fig. 1e,f ). Such observation is consistent with the results obtained from the size analyses of concentrated Van in aqueous solution with size-exclusion chromatography, dynamic light scattering and small-angle X-ray scattering [35] . The formation of the nanometer-sized Van aggregates is a result of the fact that Van easily forms noncovalent, asymmetric dimmers—mostly through multiple hydrogen bond—where the dimerization surface is on the opposite side (back) of the molecule from the ligand binding pocket [36] . Loll and co-workers [35] further asserted that collective back–back and side–side interactions between Van monomers facilitate the self-association formation of large supramolecular complex (more than six Van monomers). Their calculation also showed that the multiple noncovalent interactions engender variation in molecular conformation. Such considerably broad distribution in conformational disparity is expected to induce vastly variant intramolecular mode coupling and thus vibrational frequency shifting within individual Van monomers. As a consequence, the resultant Raman spectrum of Van-coated Ag/AAO–SERS substrates would bear huge inhomogeneous broadening. (A well-known example of such broadening caused by multiple hydrogen bonds is observed in the Raman spectrum of water. Specifically, the OH stretching mode is broadened into a huge band between 2,900 and 3,700 cm −1 ). Such broadening originates from the various configurations for Van molecules to aggregate into nanoparticles as a result of the relatively weak multiple hydrogen bonds, which is very different from the more rigid molecular architecture of the bacterial cell wall. Therefore, although the Van nanoparticles are closer to SERS substrate than the cell wall and expected to receive stronger electromagnetic enhancement, their sharp spectral features are completely smeared out by the broadening, as clearly demonstrated in Supplementary Figure S1 . The two broad Raman bands from Van-coated substrates do not present significant interference to the sensing capability of Ag/AAO–SERS substrates. This is very different from the interference produced by other functionalization agents such as antibodies, which exhibits both sharp peaks and broad background. For the Van coating, we just need to make sure the background signal produced by the Van-coating is low enough. As shown by Figure 3a , the background of the Van-coated SERS substrate alone is less than one half of that of a typical SERS spectrum of bacteria, indicating its acceptability in practical applications. As other glycopeptide antibiotics easily form aggregates as well [37] , the SERS substrates coated with those cell-wall targeted antibiotics are anticipated to easily capture bacteria with some specificity and simultaneously confer a similar featureless, broad SERS background. The bacterium-sensing capability of Van-coated Ag/AAO–SERS substrates is demonstrated by the Raman spectra of L. plantarum and E. coli ( Fig. 3b ) that exhibit substantial enhancement relative to their respective counterparts derived from pristine substrates. The dependence of the enhancement factor on the Van coverage is portrayed in Figure 2 that shows the ratio between the Raman intensity at 733 cm −1 of L. plantarum on the Van-coated substrates and that on the pristine substrates, I 733 (Van)/ I 733 (Pristine), against Van coverage. Note that the ratio reaches its maximum at a Van coverage of about 4 μg cm −2 that corresponds to an average Van thickness of ~10 nm that is just within the effective range of electromagnetic enhancement of SERS [8] . This optimal coverage reflects a compromise between the opposite developments that respond to the change in the Van coverage. On the one hand, the quantity of adhered bacteria is increased with the increased Van coverage, making more bacteria experience enhanced Raman scattering. The average distance of those attached bacteria from the SERS substrate underneath is, on the other hand, also increased, thus compelling the bacteria away from the effective range of SERS. Similarity in SERS spectra Figure 3b compares SERS spectra of bacteria acquired on pristine and Van-coated substrates. The spectra of L. plantarum on both substrates are very similar, except their distinct intensities. The positions of all the major peaks are essentially identical. Such a spectral similarity provides strong evidence to support the notion that the major sharp SERS signals originate from the same origin. (To be noted, the SERS spectrum of a Van-coated substrate without bacteria exhibits only two broad bands, as shown in Figure 3a , and, therefore, Van is not the origin of the sharp signals.) The spectra of E. coli on both substrates appear mostly similar, except in the frequency range of from 1,200 to 1,700 cm −1 . In light of the possible aggregate form of Van on the SERS substrate discussed above, the adhesion mechanism of Gram-positive bacteria on the Van-coated substrate is anticipated to be quite distinct from that of Gram-negative bacteria, owing to their differing cell envelopes. The outer membrane of the adhered E. coli may experience more conformational alternation to allow binding of Van with its interior peptidoglycan layer, leading to change in the Raman activities of certain vibrational modes. Nevertheless, such subtle difference does not alleviate the usage of such Van-coated SERS substrate for bacterial capture and detection. 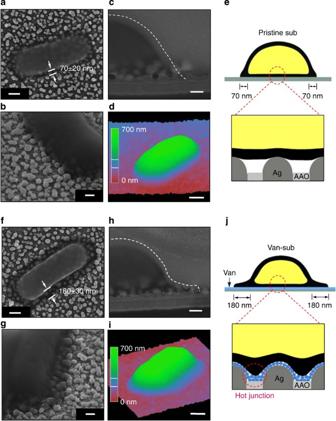Figure 4: Morphologies of cell walls of bacteria on pristine and Van-coated SERS substrates. (a–e) Pristine and (f–j) Van-coated SERS substrates. (a,f) Top-view SEM images (scale bar, 200 nm). (b,g) Oblique-angle-view SEM images (viewing angle of 52°; scale bar, 100 nm). (c,h) Crosssection-view SEM images (sample prepared by FIB dissection, scale bar, 100 nm). (d,i) 3D AFM images. (e,j) Schematics showing the cross-section of bacteria on two kinds of substrates (scale bar, 300 nm). Bacteria cell-wall deformation Figure 4 shows the deformation in bacteria's cell wall due to their adhesion onto pristine and Van-coated Ag/AAO–SERS substrates, respectively. The SEM top-view ( Fig. 4a,f ) and prospective-view ( Fig. 4b,g ) images show that a significant portion of the cell wall is stretched and forms a thin rim attaching to the substrate. The range of the stretch is 70 nm and 180 nm for pristine and Van-coated substrates, respectively. Both the oblique-view ( Fig. 4b,g ) SEM images and the atomic force microscope (AFM) images ( Fig. 4d,i ) show that surface topography of the stretched rim has a slop, starting from 160 (100) nm and terminating at 70 (30) nm above the pristine (Van-coated) substrate surface. In other words, the rims of bacteria on Van-coated substrate are stretched 2.5 times further and become 2.3 times thinner along the outermost edge. The larger and thinner stretched rim indicates that the bacterial cell wall is deformed to maximize its favourable interaction with the densely distributed Van nanoparticles, thus augmenting its effective adhesive force to the substrate. Figure 4: Morphologies of cell walls of bacteria on pristine and Van-coated SERS substrates. ( a – e ) Pristine and ( f – j ) Van-coated SERS substrates. ( a , f ) Top-view SEM images (scale bar, 200 nm). ( b , g ) Oblique-angle-view SEM images (viewing angle of 52°; scale bar, 100 nm). ( c , h ) Crosssection-view SEM images (sample prepared by FIB dissection, scale bar, 100 nm). ( d , i ) 3D AFM images. ( e , j ) Schematics showing the cross-section of bacteria on two kinds of substrates (scale bar, 300 nm). Full size image Focused ion beam (FIB) was used to dissect the bacteria to reveal their cross-section and interface with the underlying substrate. The SEM images ( Fig. 4c,h ) of the cross-sections again demonstrate the existence of a larger stretched rim on the cell wall of bacteria on the Van-coated substrate. On the basis of the above observations, we sketch the cell-wall deformation of bacteria on pristine and Van-coated Ag/AAO–SERS substrates in Figure 4e,j, respectively. The area covered by the rim constitutes 20% (50%) of the total area on the cell envelope in contact with the pristine (Van-coated) substrate. The 30% increase in the contact area is qualitatively consistent with the observed increase in the SERS signal obtained on the Van-coated substrate. However, it cannot account for the 400–500% signal enhancement. We have to resort to some other origin for the one order of magnitude discrepancy. Close comparison of the stretched rims in the prospective-view images ( Fig. 4b,g ) of bacteria on pristine and Van-coated substrates reveal a subtle difference in their contact with the underlying Ag-nanoparticle arrays, which could help resolve the discrepancy. The cell wall on the former partially sits on the top surface of the Ag nanoparticles, while that on the latter penetrates into the gap between adjacent Ag nanoparticles. Insets of Figure 4e,j depict schematically the characteristic difference between the two cell-wall/substrate interfaces. It appears that the Van coating provides the extra force to pull the cell wall towards the substrate and fill up the gaps between the nanoparticles. As the gaps are the 'hot junctions' for the electromagnetic enhancement of Raman scattering and such enhancement decays almost exponentially with respect to the molecule–substrate separation [38] , one can expect the pulling of a small portion of the cell wall closer to the hot junctions could lead to a very large enhancement in the Raman signal. This scenario could explain the observed 400–500% increase in the SERS signal of bacteria on Van-coated substrates. Although the cell walls of E. coli on a pristine substrate do not show a stretched rim ( Supplementary Fig. S2a ), that on a Van-coated substrate clearly exhibit one as wide as ~150 nm ( Supplementary Fig. S2b ). The oblique-angle-view SEM images ( Supplementary Fig. S2c,d ) moreover demonstrate that the cell wall of the bacteria closely follow the corrugation of the Van-coated substrate, indicating that the Van coating on the surface of the Ag/AAO–SERS substrate also adheres strongly to the cell wall of Gram-negative bacteria. The pulling of the bacterial cell wall closer to the hot junctions between Ag-nanoparticles could also be evoked to account for the several-fold increase in the SERS signal of E. coli on a Van-coated substrate ( Fig. 3b ). The stronger binding between a Van-coated substrate and a bacterium relies on the interaction between Van and the substrate as well as that between Van and the cell wall. We can gain some insights about the interaction by comparing the surface morphology of pristine ( Fig. 1e ) and Van-coated ( Fig. 1f ) substrates. Ag nanoparticles evidently protrude above alumina nanochannels with round top-surfaces on the pristine substrate, while they are decorated by many Van-nanoparticles with few nanometers in diameter on the Van-coated substrate. The finding suggests that the Van nanoprticles would serve as the anchors to bind the cell wall to the substrate surface. The molecular origin of the binding between bacteria and Van could be traced back to the hydrogen bonds (N-H...O) between the L -Lys- D -Ala- D -Ala (or D -Lac) of the peptidoglycan of the cell wall and the carbonyl or amine groups on the Van, as shown in Supplementary Figure S3 (refs 23 , 24 , 31 ). Conceptually, a Van-coating layer with such multiple sites of hydrogen bonds is similar to a velcro tape. Its stickiness depends almost exponentially on the density of the bonding sites. This type of behaviour is consistent with the observation that the bacterial sticking probability increases by ~1,000-fold as the coverage of the Van coating increases by only a factor of 50 ( Fig. 2 ). The energetics involved in the enhanced sticking can be carried out by estimating the energy needed to reduce the height of bacteria on the pristine substrate to that on the Van-coated substrate (a few tens of nanometers shown in Fig. 4c,h ). According to the previous studies [39] , [40] , it would require ~100 μN to reduce the height of bacteria by a few tens of nanometers. Therefore, the extra strain energy stored in the bacteria cell wall on the Van-coated substrate is ~10 −11 J, which is comparable to the energy associated with the N-H...O hydrogen bonds between peptidoglycan of the cell wall and Van. Furthermore, Axelsen's group [37] through elaborate simulation showed that the gain of configuration entropy, owing to the collectivity between the ligand binding and the dimerization in Van, would further the stereo-specific binding and also stabilize the aggregation. Accordingly, such nanometer-sized Van aggregates might serve two functions in the context of seizing bacteria. First, the multiple ligand-binding packets and the cooperative interaction within the Van nanoparticle would strengthen the binding with bacteria. Second, their nanometer-sized dimension would allow for thorough filling of any possible gap between the round, deformed bacterial surface and the corrugated, rigid surface of the Ag/AAO substrate, thus providing optimal binding between them. In a microscopic perspective, a recent solid-state NMR study showed that a great portion of the peptides present in the cell-wall peptidoglycan is uncross-linked [41] . Such uncross-linked peptides likely represent the binding entities that can easily permeate into the ligand-binding pockets within the Van aggregates. This picture is supported by the recently revealed three-dimensional structural model of peptidoglycan [42] , as pointed out by Loll et al . [35] Capture bacteria from human blood As a test for the potential clinical applications of the functionalized Ag/AAO–SERS substrates, capturing and sensing L. plantarum that were spiked into human blood were conducted [26] . 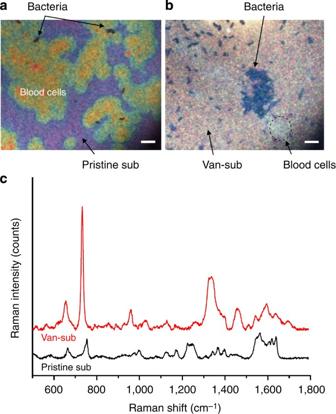Figure 5: Optical microscope images and SERS spectra of bacteria and blood cells captured using pristine and Van-coated substrates from bacterium-spiked human blood sample. Preferential capturing of (a) blood cells (bright-yellow area) on a pristine substrate and (b) bacteria (L. plantarum, dark green area) on a Van-coated substrate. (c) SERS spectrum of bacteria spiked into human blood on a pristine substrate (a) and that on a Van-coated substrate (b) (all scale bars, 5 μm). The results shown in Figure 5 and Supplementary Table S1 indicate that the sticking probability of blood cells (that is, white blood cells, red blood cells, platelets and so on) on pristine substrates ( Fig. 5a ) is 60 times higher than that on Van-coated substrates. On the contrary, the sticking probability of bacteria on pristine substrates is 300-fold lower than that on Van-coated substrates ( Fig. 5b ). The SERS spectrum of the bacteria captured from blood onto a Van-coated substrate ( Fig. 5c ) appears similar to that of bacteria captured from water onto a Van-coated substrate ( Fig. 3b ). In contrast, the SERS spectrum acquired from the pristine substrate covered by blood cells exhibits drastically different vibrational signatures that are essentially the same as that of blood cells from an un-spiked blood sample ( Supplementary Fig. S4 ), indicating that the pristine substrate is overwhelmed by the blood cells and other constituents in the blood. To some extent, such specific binding between Van and bacteria is within our expectation, since Van—being one of the most effective antibiotic—is synthetically optimized to target bacteria specifically and also to minimize any possible attack to normal body cells. In addition to their specific bacterium-binding capability, the Van-coated substrates also provide similar SERS spectra (not shown) of bacteria captured from human blood. Therefore, Van functionalization is an effective means not only to reduce the adhesion of blood cells and biomolecules in the blood onto the Ag/AAO–SERS substrate but also to capture bacteria for the follow-up SERS sensing process. Figure 5: Optical microscope images and SERS spectra of bacteria and blood cells captured using pristine and Van-coated substrates from bacterium-spiked human blood sample. Preferential capturing of ( a ) blood cells (bright-yellow area) on a pristine substrate and ( b ) bacteria ( L. plantarum , dark green area) on a Van-coated substrate. ( c ) SERS spectrum of bacteria spiked into human blood on a pristine substrate ( a ) and that on a Van-coated substrate ( b ) (all scale bars, 5 μm). Full size image Differentiate VSE and VRE To be noted, both E. coli and L. plantarum used for demonstrating the bacterium-capturing capability of the Van-coated SERS substrates are intrinsically resistant to Van. Van is known to attack most Gram-positive bacteria by disrupting the synthesis of their cell walls, although it is not an effective drug against Gram-negative bacteria owing to their different cell synthesis mechanism. However, Lactobacillus is an exceptional Gram-negative bacterium because of its different cell-wall structure [43] . The development of Van resistance is often attributed to the reduced number of hydrogen bonds with the altered peptidoglycan in the cell wall of the mutated bacteria [44] . Given the sensitive bacterium-binding ability of the Van-coated substrate, it is therefore interesting to ask whether the Van-coated substrate can also be used to test the Van suceptibility of certain strain of Gram-positive bacteria. 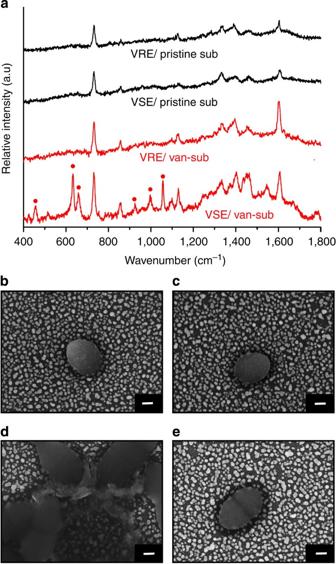Figure 6: SEM images and SERS spectra of VSE and VRE on pristine and Van-coated SERS substrates. (a) SERS spectra of VSE and VRE on a Van-coated substrate and pristine substrate. SEM images of (b) VSE on a pristine substrate, (c) VRE on a pristine substrate, (d) VSE on a Van-coated substrate and (e) VRE on a Van-coated substrate (all scale bars, 200 nm). Figure 6a shows SERS spectra of Van-susceptible Enterococcus (VSE) and Van-resistant Enterococcus (VRE) on the pristine and Van-coated SERS substrates. Note that both SERS spectra of VSE and VRE on pristine substrates are essentially indistinguishable whereas those on Van-coated substrates are drastically different. Specifically, several extra peaks (labelled by dots) appear distinctively on the SERS spectrum of VSE on the Van-coated substrate, whereas that of VRE remains very similar to the spectra of both VRE and VSE on pristine substrates. Therefore, the results demonstrate the feasibility of using the Van-coated substrate to test the drug susceptibility of certain strain of Gram-positive bacteria. Figure 6: SEM images and SERS spectra of VSE and VRE on pristine and Van-coated SERS substrates. ( a ) SERS spectra of VSE and VRE on a Van-coated substrate and pristine substrate. SEM images of ( b ) VSE on a pristine substrate, ( c ) VRE on a pristine substrate, ( d ) VSE on a Van-coated substrate and ( e ) VRE on a Van-coated substrate (all scale bars, 200 nm). Full size image To find some clue for the origin of the extra peaks appearing on the SERS spectrum of VSE on a Van-coated substrate, SEM images of VSE and VRE on both substrates were acquired and are shown in Figure 6b–e . Images of VSE and VRE on a pristine substrate appear identical ( Fig. 6b,c ), as expected from their identical SERS spectra. In contrast, on Van-coated substrates, the cell walls of many VSE are disrupted and certain secretion is clearly observed ( Fig. 6d ) whereas that of VRE remain intact ( Fig. 6e ). We therefore propose that the extra peaks in the SERS spectrum of VSE on a Van-coated substrate is originated from the secretion. Our observations are qualitatively consistent with the notion that Van can attack the cell wall of VSE through the strong five-point hydrogen bonding to its NAG/NAM-peptide linker, but cannot effectively bind VRE because of the 1,000-fold decrease in the affinity of Van to the mutated peptide linker [27] . As to the question regarding the detailed mechanism of the reaction of the VSE strain to the Van-coated substrate, its answer entails more elaborate investigations in the possible biochemical processes following the Van-peptide interaction. The discovery that Van-coating can add bacterium-capturing function to the Ag/AAO–SERS substrates without introducing significant interference to their SERS sensing capability is completely unexpected, because one would expect the SERS of Van to exhibit sharp, rather than broad, spectral features that can be easily treated by background subtraction. Although such a spectral broadening could be qualitatively explained by a mechanism based on hydrogen-bond mediated aggregate nature of Van, more researches are certainly needed to clarify its detailed mechanism and the seemingly low SERS response of the Van-coating. Similarly, the observed 400–500% increase in the SERS signal of captured bacteria is counterintuitive because the Van-coating should increase the separation between the cell wall and thus reduce the SERS signal. Such a signal enhancement could be qualitatively understood in terms of the improved penetration of the bacteria cell wall into the gaps between the Ag nanoparticles on the SERS substrates caused by the Van-coating. However, the revelation of the binding mechanism involved demands further studies. The demonstration to capture bacteria in water or human blood onto a microscopic area of Ag/AAO–SERS substrate with Van-coating is clearly a major step towards the development of a high speed and sensitivity nanotechnology platform that has high potential to capture/detect bacteria in clinical or environmental samples. This nanotechnology platform is expected to have much better reproducibility than the conventional approaches such as mixing nanoparticles with bacteria because of the extremely high uniformity and density of Ag-nanoparticles on the Ag/AAO–SERS (For more information about the reproducibility, see Supplementary Figs S5 and S6 as well as refs 4 and 21 ). In principle, other glycopeptides with different hydrogen bonding configurations to target other microorganisms such as virus could be employed to coat the Ag/AAO–SERS substrates and create a nano-biotechnology platform for the fabrication of multifunctional biochips. Vancomycin coating of SERS substrates Ag/AAO–SERS substrates consisting of arrays of Ag-nanoparticles partially embedded in AAO nanochannels were fabricated according to the methods described previously [4] , [21] . To coat Van, substrates (1×1 cm 2 ) were immersed in the various concentration (100 mM–80 μM) of Van hydrochloride (Sigma) aqueous solution for 1 h, and then dried in the air for 12 h. UV-Visible spectrometry (Metertech, SP-8001) was employed to measure the amount of Van in the solution before and after the coating process. The difference in the extracted absorbance data determined the amount of Van covered on the substrate, which was then used to estimate the average thickness of Van coating, assuming the density of Van is 1.65 g cm −3 . Bacteria growth and sample preparation Escherichia coli ( E. coli , ATCC 11775), Lactobacillus plantarum ( L. Plantarum , ATCC 8014), vancomycin-susceptible Enterococcus faecails (VSE, ATCC 29212), and vancomycin-resistant Enterococcus faecails (VRE, ATCC 51299) were purchased from Bioresouce Collection and Research Center. Both bacteria were cultivated for 16 h at 37 °C on Nutrient and MRS agar base, respectively. After sub-culturing, single colonies were collected using sterile plastic inoculating loops. Bacteria were then suspended in 5 ml of Nutrient and MRS broth respectively, grown for a further 14 h and then subcultured until OD 600 reached ~0.5. Bacteria thus obtained were used for all the experiments. For SERS measurements, bacteria were washed and centrifuged three times with deionized water and re-suspended in water again. Typically, 1 ml of the sample solution was placed on a SERS substrate and then stored in an orbital shaking incubator (OSI500R, TKS) operated at 120 r.p.m. and 37 °C for 1 h. The sample was washed five times with water before the Raman measurement. Characterization Raman measurements were performed with a commercial Raman microscope (HR800, Horiba). A HeNe laser, emitting at 632.8 nm, served as the excitation source. The laser beam was focused onto the sample through a X50 objective lens. The backward radiation was collected by the same lens and was then delivered to an 80-cm spectrograph equipped with a liquid-nitrogen-cooled charge-coupled device for spectral analysis. Raman spectra were collected in the frequency ranging from 400 to 1,800 cm −1 with a typical acquisition time of 60 s. (By using a X100 water-immersion objective lens on the apparatus, high-quality single-bacteria SERS spectrum are routinely obtained in 1 to 3 s., as demonstrated in ref. 21 ). A background subtraction program, based on the algorithm proposed by Miroslav's group [45] , was developed to process the obtained Raman spectra. The numbers of bacteria and blood cells were counted with a commercial software (Scanning Probe Image Processor). Scanning electron microscopic examination and needed sample preparation were conducted with a DualBeam FIB/SEM system (Nova 600, FEI). Surface morphology characterization of bacteria and substrates was performed with an atomic force microscopic system (MMAFM-2, Digital Instrument). How to cite this article: Liu, T-Y. et al . Functionalized arrays of Raman-enhancing nanoparticles for capture and culture-free analysis of bacteria in human blood. Nat. Commun. 2:538 doi: 10.1038/ncomms1546 (2011).